Early adipogenesis is regulated through USP7-mediated deubiquitination of the histone acetyltransferase TIP60 Transcriptional coregulators, including the acetyltransferase Tip60, have a key role in complex cellular processes such as differentiation. Whereas post-translational modifications have emerged as an important mechanism to regulate transcriptional coregulator activity, the identification of the corresponding demodifying enzymes has remained elusive. Here we show that the expression of the Tip60 protein, which is essential for adipocyte differentiation, is regulated through polyubiquitination on multiple residues. USP7, a dominant deubiquitinating enzyme in 3T3-L1 adipocytes and mouse adipose tissue, deubiquitinates Tip60 both in intact cells and in vitro and increases Tip60 protein levels. Furthermore, inhibition of USP7 expression and activity decreases adipogenesis. Transcriptome analysis reveals several cell cycle genes to be co-regulated by both Tip60 and USP7. Knockdown of either factor results in impaired mitotic clonal expansion, an early step in adipogenesis. These results reveal deubiquitination of a transcriptional coregulator to be a key mechanism in the regulation of early adipogenesis. Adipogenesis, the differentiation of fibroblast-like mesenchymal stem cells into adipocytes, is studied extensively for its importance in the regulation of energy metabolism. A widely accepted adipogenesis model is the 3T3-L1 cell line, which can efficiently be differentiated into mature adipocytes by hormonal stimulation under experimental conditions [1] . During adipogenesis, cells are first growth-arrested, subsequently treated with differentiation inducers to synchronously re-enter the cell cycle and undergo mitotic clonal expansion (MCE) and finally exit the cell cycle to undergo terminal differentiation. MCE is a prerequisite for 3T3-L1 differentiation [2] , underscoring the intimate relationship between cell cycle regulation and differentiation in this model system for adipogenesis. Adipogenesis is regulated by a cascade of transcription factors, including the CCAAT enhancer-binding proteins and Peroxisome proliferator activator receptor γ (PPARγ) [3] . Post-translational modifications (PTMs), such as phosphorylation, acetylation, sumoylation and ubiquitination, can regulate the transcriptional output of these transcription factors (reviewed in van Beekum et al . [4] and Nerlov [5] ). PTM can affect various aspects of transcription factor function including subcellular localization, protein stability and interactions with transcriptional coregulators. Interestingly, several transcriptional coregulators are also subject to PTM, offering the possibility to fine-tune transcriptional activity [6] . A clear example of this is the coactivator SRC-3, which is essential for adipogenesis in vitro and in vivo [7] , [8] . SRC-3 is subject to phosphorylation, methylation, acetylation and ubiquitination, regulating its subcellular localization, activity and stability (reviewed in Hans et al . [6] and York and Malley [9] ). Another example of a coregulator undergoing PTM is Tip60 (HIV-1 Tat-interacting protein 60), a member of the MYST family of acetyltransferases [10] . Tip60 is the catalytic subunit of the highly conserved NuA4 acetyltransferase complex, which has a key role in transcription regulation and DNA damage repair. Tip60 acetylates histone proteins (H4, H2A, H2A.X and H2A.Z) and various transcription factors, thereby activating or repressing transcription. The Tip60 complex can also modify chromatin around DNA double-stranded breaks to support repair, demonstrating an additional important cellular function [10] . Its role in these two fundamental cellular processes may explain the embryonic lethality observed in Tip60 knockout mice [11] , [12] and early pupal lethality after Tip60 depletion in Drosophila melanogaster [13] . Similar to SRC-3, Tip60 can undergo multiple PTM, including phosphorylation [14] , sumoylation [15] and ubiquitination [16] . Phosphorylation and sumoylation regulate the acetyltransferase activity of Tip60 (refs 14 , 15 ), and ubiquitination results in degradation of the protein by the proteasome [16] . Whereas PTM, therefore, presents an important mechanism to regulate the activity of transcriptional coregulators such as SRC-3 and Tip60, demodification may have an equally important role in balancing the transcriptional output. However, current knowledge on enzymes which can, for example, deubiquitinate coregulator proteins is very limited. Recently, we found Tip60 to be essential for the differentiation of 3T3-L1 adipocytes [17] . As Tip60 protein levels, but not mRNA levels, are upregulated during adipogenesis [17] , [18] , and as Tip60 can be degraded by the proteasome [16] , [19] , these findings suggest that the Tip60 protein may be stabilized through deubiquitination during adipogenesis. Here we describe the identification of USP7 (also known as HAUSP) as an essential deubiquitinase in adipogenesis. Tip60 can be deubiquitinated by USP7 in intact cells and in vitro , qualifying Tip60 as a direct substrate of USP7. RNA interference (RNAi)-mediated knockdown of USP7 and Tip60 affects a common set of target genes, which are predominantly involved in cell cycle regulation. In agreement with this, RNAi-mediated knockdown of USP7 and Tip60 impairs MCE. Taken together, our findings reveal deubiquitination of a transcriptional coregulator as a novel mechanism in the regulation of early adipogenesis. The deubiquitinase USP7 is essential for adipogenesis Expression of the Tip60 protein, but not mRNA, increases during the first stages of 3T3-L1 differentiation ( Fig. 1a (ref. 17 )), suggesting that this protein may be regulated by deubiquitination during adipogenesis. To identify specific dominant deubiquitinating enzyme (DUB) activities during adipogenesis, we made use of an HA-tagged probe that covalently binds active DUBs [20] . Incubation of 3T3-L1 lysates with this probe followed by western blotting (WB) with an HA antibody revealed only two major DUB activities during adipogenesis ( Fig. 1b ), whereas 293 T cells ( Fig. 1b ) and other cell types [21] display multiple activities. Interestingly, the increase in enzymatic activity of the two dominant DUBs during adipogenesis coincided with increased Tip60 protein expression (day 2; Fig. 1a,b ). On the basis of the molecular weights (~130 and ~37 kD), we predicted that the high molecular weight activity may present USP7 (also known as HAUSP), a DUB best known for its involvement in the p53-mdm2 pathway [22] . Immunoprecipitation of active DUBs through the HA-tagged probe from mature 3T3-L1 adipocytes followed by WB with anti-USP7 antibodies showed that the high molecular weight DUB activity in mature adipocytes was indeed USP7 ( Fig. 1c ). We recently identified the low molecular weight activity as the cytoplasmic DUB UCHL3 (ref. 23 ). 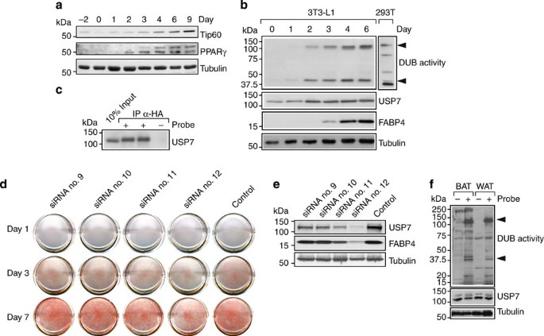Figure 1: USP7 is essential for adipogenesis. (a) Mouse 3T3-L1 preadipocytes were differentiated into mature adipocytes, and samples were taken at different time points during differentiation. Protein expression levels of Tip60 and PPARγ were determined using western blot analysis. Original immunoblot images forFig. 1are shown inSupplementary Fig. S8. (b) 3T3-L1 cells were differentiated and cells were lysed at different time points. Cells lysates were incubated with a vinyl methyl ester HA-Ub probe to covalently tag active DUBs. DUB activity was detected using western blotting (anti-HA antibody). Protein expression levels of USP7 were determined using western blot analysis. As a control for differentiation, FABP4 protein levels were analysed. (c) Cell lysates of differentiated 3T3-L1 cells (day 6) were incubated with or without HA-Ub probe; DUB activities were immunoprecipitated (anti-HA agarose) and USP7 was detected using western blotting. Note the difference in mobility between unmodified USP7 (input lane) and USP7 covalently bound to the DUB probe. (d) 3T3-L1 cells, transfected with either control or USP7 siRNA oligonucleotides, were subjected to differentiation conditions. On day 0, 3 or 6 of differentiation, cells were fixed and stained for triglycerides using Oil-red-O. Pictures are representative for three independent experiments. (e) 3T3-L1 cells were transfected with either control or USP7 siRNA oligonucleotides during differentiation as described under (d). Cell lysates were subjected to western blot analysis, using antibodies against USP7, FABP4 and tubulin. (f) Mouse BAT and WAT were collected, tissues were lysed and DUB activity was determined as described under (b). Figure 1: USP7 is essential for adipogenesis. ( a ) Mouse 3T3-L1 preadipocytes were differentiated into mature adipocytes, and samples were taken at different time points during differentiation. Protein expression levels of Tip60 and PPARγ were determined using western blot analysis. Original immunoblot images for Fig. 1 are shown in Supplementary Fig. S8 . ( b ) 3T3-L1 cells were differentiated and cells were lysed at different time points. Cells lysates were incubated with a vinyl methyl ester HA-Ub probe to covalently tag active DUBs. DUB activity was detected using western blotting (anti-HA antibody). Protein expression levels of USP7 were determined using western blot analysis. As a control for differentiation, FABP4 protein levels were analysed. ( c ) Cell lysates of differentiated 3T3-L1 cells (day 6) were incubated with or without HA-Ub probe; DUB activities were immunoprecipitated (anti-HA agarose) and USP7 was detected using western blotting. Note the difference in mobility between unmodified USP7 (input lane) and USP7 covalently bound to the DUB probe. ( d ) 3T3-L1 cells, transfected with either control or USP7 siRNA oligonucleotides, were subjected to differentiation conditions. On day 0, 3 or 6 of differentiation, cells were fixed and stained for triglycerides using Oil-red-O. Pictures are representative for three independent experiments. ( e ) 3T3-L1 cells were transfected with either control or USP7 siRNA oligonucleotides during differentiation as described under ( d ). Cell lysates were subjected to western blot analysis, using antibodies against USP7, FABP4 and tubulin. ( f ) Mouse BAT and WAT were collected, tissues were lysed and DUB activity was determined as described under ( b ). Full size image To address the relevance of USP7 in adipogenesis, the expression of this protein was reduced using siRNA-mediated knockdown. Adipogenesis was inhibited by siRNA oligonucleotides against USP7, as illustrated by triglyceride staining with Oil-red-O ( Fig. 1d ) and FABP4 expression ( Fig. 1e ) on day 6 of differentiation. The degree of inhibition correlated with the reduction in USP7 protein expression, with oligonucleotide no. 12 being the most efficient and oligonucleotide no. 11 displaying a partial effect. Importantly, USP7 represented not only a major DUB activity in the 3T3-L1 cell culture system ( Fig. 1b ) but also in mouse white and brown adipose tissues (WAT and BAT, respectively; Fig. 1f ). Together, these data qualify USP7 as a major and essential deubiquitinating enzyme in mature adipocytes. USP7 interacts with and deubiquitinates Tip60 As Tip60 can be polyubiquitinated [16] , [19] and as USP7 activity is upregulated during adipogenesis ( Fig. 1 ), we investigated whether Tip60 may be a direct USP7 deubiquitination substrate. We therefore first examined the interaction between these two proteins. Cells were cotransfected with HA-tagged Tip60 and myc-tagged USP7, followed by immunoprecipitation. As shown in Fig. 2a , Tip60 co-immunoprecipitated with myc-tagged USP7 and vice versa . As controls, immunoprecipitations were performed on cell lysates in which neither or only one of the proteins was present. No co-immunoprecipitations were observed in these cases ( Fig. 2a ) nor did USP7 co-immunoprecipitate with PPARγ ( Supplementary Fig. S1 ). More detailed protein–protein interaction studies revealed that deletion of the N-terminal region, or mutation of the chromodomain located within this region (F47A/Y50A), severely inhibited the interaction ( Fig. 2b ). Mutation of the zinc finger (C263A) or the NR box (L492A/L493A), domains that have been implicated in interactions with other proteins previously [10] , had little effect ( Fig. 2b ). While being essential, the N-terminus of Tip60 is not sufficient for USP7 binding (for example, 1–286 and 1–488 constructs), suggesting that Tip60 interacts with USP7 through multiple domains. GST-pull-down experiments confirmed the Tip60–USP7 interaction in vitro ( Fig. 2c ). 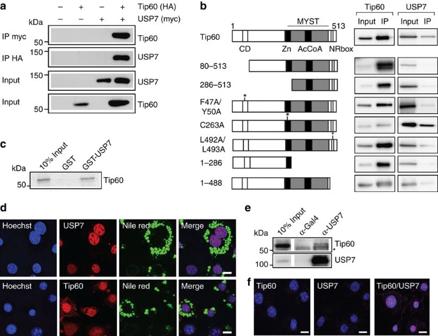Figure 2: USP7 interacts with Tip60. (a) Myc-tagged USP7 and HA-tagged Tip60 were expressed either alone or together in HEK293T cells. After lysis, USP7 and Tip60 were immunoprecipitated with anti-myc and anti-HA antibodies, respectively. Immunoreactive proteins were detected on western blots with anti-HA and anti-myc antibodies. Original immunoblot images forFig. 2are shown inSupplementary Fig. S9. (b) Myc-tagged USP7 and various HA-tagged Tip60 proteins (depicted schematically on the left) were expressed together in HEK293T cells. Immunoprecipitations were performed as described under (a). (c) Bacterially expressed and purified GST-USP7 protein was incubated with [35S]-labelled Tip60 protein. Samples were subjected to SDS–PAGE, and labelled proteins were visualized using fluorography. (d) Representative confocal microscopy images of 3T3-L1 adipocytes. Endogenous Tip60 and USP7 (both red) were visualized utilizing specific antibodies; differentiated cells were identified with Nile Red (green); and Hoechst was used to visualize the nuclei (blue). Scale bar, 10 μm. (e) Interaction between endogenous Tip60 and USP7 proteins in differentiated 3T3-L1 cells. USP7 was immunoprecipitated from cell lysates of differentiated 3T3-L1 cells (day 6). Immunoreactive proteins were detected on western blots with anti-USP7 and anti-Tip60 antibodies. As a control, an irrelevant antibody was used (anti-Gal4 antibody). An aspecific band is indicated (*). (f) Tip60–USP7 was visualized in 3T3-L1 adipocytes using anin situPLA. Cells were fixed and protein–protein interactions were visualized utilizing anti-Tip60 and anti-USP7 antibodies. Punctate staining (red) indicates a Tip60–USP7 interaction as detected by the assay. Hoechst was used to visualize the nuclei (blue). Scale bar, 10 μm. Figure 2: USP7 interacts with Tip60. ( a ) Myc-tagged USP7 and HA-tagged Tip60 were expressed either alone or together in HEK293T cells. After lysis, USP7 and Tip60 were immunoprecipitated with anti-myc and anti-HA antibodies, respectively. Immunoreactive proteins were detected on western blots with anti-HA and anti-myc antibodies. Original immunoblot images for Fig. 2 are shown in Supplementary Fig. S9 . ( b ) Myc-tagged USP7 and various HA-tagged Tip60 proteins (depicted schematically on the left) were expressed together in HEK293T cells. Immunoprecipitations were performed as described under ( a ). ( c ) Bacterially expressed and purified GST-USP7 protein was incubated with [ 35 S]-labelled Tip60 protein. Samples were subjected to SDS–PAGE, and labelled proteins were visualized using fluorography. ( d ) Representative confocal microscopy images of 3T3-L1 adipocytes. Endogenous Tip60 and USP7 (both red) were visualized utilizing specific antibodies; differentiated cells were identified with Nile Red (green); and Hoechst was used to visualize the nuclei (blue). Scale bar, 10 μm. ( e ) Interaction between endogenous Tip60 and USP7 proteins in differentiated 3T3-L1 cells. USP7 was immunoprecipitated from cell lysates of differentiated 3T3-L1 cells (day 6). Immunoreactive proteins were detected on western blots with anti-USP7 and anti-Tip60 antibodies. As a control, an irrelevant antibody was used (anti-Gal4 antibody). An aspecific band is indicated (*). ( f ) Tip60–USP7 was visualized in 3T3-L1 adipocytes using an in situ PLA. Cells were fixed and protein–protein interactions were visualized utilizing anti-Tip60 and anti-USP7 antibodies. Punctate staining (red) indicates a Tip60–USP7 interaction as detected by the assay. Hoechst was used to visualize the nuclei (blue). Scale bar, 10 μm. Full size image Next, we examined the interaction between the endogenous Tip60 and USP7 proteins in 3T3-L1 adipocytes. As both cytoplasmic and nuclear localizations of Tip60 (ref. 10 ) and USP7 (ref. 22 ) have been reported, we first investigated the localization of the proteins in differentiated 3T3-L1 cells. For this immunofluorescent staining of Tip60 and USP7 was combined with fluorescent staining for intracellular lipid droplets (Nile red) to mark differentiating cells. Tip60 and USP7 both displayed nuclear localization in mature 3T3-L1 adipocytes, whereas Tip60 was also present in the cytoplasm ( Fig. 2d ). To further validate the Tip60–USP7 interaction, we performed endogenous co-immunoprecipitation experiments in these cells. Tip60 could be detected after immunoprecipitation with an antibody against USP7 but not with an irrelevant antibody (Gal4) ( Fig. 2e ). To confirm this direct association between endogenous USP7 and Tip60, an in situ proximity ligation assay (PLA) was performed in 3T3-L1 adipocytes (Methods). As a PLA signal can only be obtained when the proteins of interest are in extremely close proximity, this technique enables the detection of direct protein–protein interactions in cells [24] , [25] . Association between USP7 and Tip60 was observed and this interaction was localized specifically to the nucleus ( Fig. 2f ). Undifferentiated 3T3-L1 cells, as identified by the lack of PPARγ expression, displayed no PLA signal ( Supplementary Fig. S2 ). To further examine the role of USP7 in regulating Tip60 protein expression levels, we tested whether USP7 could directly deubiquitinate Tip60 and thereby increase Tip60 protein levels. We first confirmed that Tip60 can be ubiquitinated by expressing Tip60 together with histidine-tagged ubiquitin in cells, followed by treatment with the proteasome inhibitor MG132. Purification of histidine-tagged proteins followed by WB with an antibody directed against Tip60 revealed high molecular weight species of Tip60, indicative of polyubiquitination ( Fig. 3a ). Mutation of all seven lysine residues in ubiquitin (7KR), which blocks polybranching of ubiquitin, prevented formation of most of the modified Tip60 forms, confirming that Tip60 is indeed polyubiquitinated ( Fig. 3a ). To identify which of the 41 lysine residues in Tip60, which are all highly conserved in evolution, were ubiquitinated, we isolated ubiquitinated Tip60 from cells, subjected the protein to digestion with several proteases ( Supplementary Table S1 ) and identified ubiquitinated sites using mass spectrometry (total coverage 74%; 36 out of 41 lysines covered). We found five high confidence ubiquitin sites and one site with lower confidence ( Fig. 3b and Supplementary Table S1 ). Substitution of these six lysines by arginines did not significantly alter Tip60 ubiquitination levels ( Supplementary Fig. S3 ), suggesting that the protein harbours additional unidentified ubiquitination sites or that Tip60 ubiquitination is promiscuous, as observed in other proteins ((ref. 21 ) and references therein). Mutation of all 41 lysine residues into arginine residues in the Tip60 protein, however, completely ablated polyubiquitination ( Fig. 3c ). We therefore conclude that Tip60 can be polyubiquitinated on multiple lysine residues. 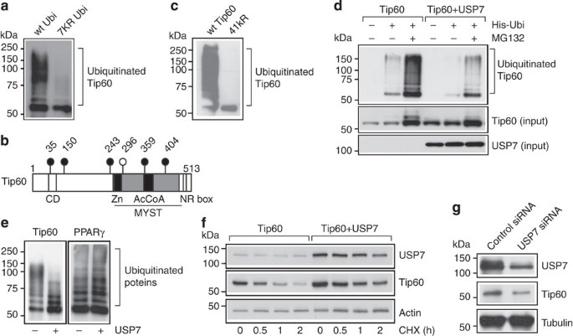Figure 3: USP7 deubiquitinates Tip60. (a) HEK293T cells were transfected with HA-tagged Tip60 expression construct together with wild-type or 7KR mutant histidine-tagged ubiquitin (His-ubi) expression construct and treated with MG132 (3 μM). Ubiquitinated proteins were isolated using Ni-NTA precipitation and ubiquitinated Tip60 was detected using western blotting (anti-HA antibody). Original immunoblot images forFig. 3are shown inSupplementary Fig. S10. (b) Schematic representation of the five high confidence (filled circles) and one lower confidence (open circle) ubiquitination sites in Tip60 identified using MS/MS. (c) HEK293T cells were transfected with wild-type HA-tagged Tip60 expression construct or the 41 KR mutant together with histidine-tagged ubiquitin (His-ubi) and treated with MG132 (3 μM). Ubiquitinated Tip60 was detected as described underb. (d) HEK293T cells were transfected with HA-Tip60 expression vector with or without myc-USP7 expression vector and with or without his-tagged ubiquitin expression vector in the absence or presence of MG132, as indicated. Cells were lysed, ubiquitinated proteins were isolated by Ni-NTA purification and immunoreactive proteins were detected on western blots by anti-HA, anti-Tip60 and anti-myc antibodies. (e) Ubiquitinated HA-Tip60 and HA-PPARγ were produced as described ina, eluted from the Ni-NTA beads with imidazole and incubated with recombinant USP7 enzyme. Tip60 and PPARγ were detected using western blot analysis (anti-HA antibody). (f) HA-Tip60 expression vector was cotransfected with empty vector or USP7 expression vector in 911 cells. Cells were treated with cycloheximide (30 ng ml−1), collected at different time points and subjected to western blot analysis. (g) Mature 3T3-L1 adipocytes were subjected to RNAi-mediated knockdown with control or USP7-specific oligonucleotides. Cell lysates were subjected to western blot analysis using antibodies against USP7, Tip60 and tubulin. Figure 3: USP7 deubiquitinates Tip60. ( a ) HEK293T cells were transfected with HA-tagged Tip60 expression construct together with wild-type or 7KR mutant histidine-tagged ubiquitin (His-ubi) expression construct and treated with MG132 (3 μM). Ubiquitinated proteins were isolated using Ni-NTA precipitation and ubiquitinated Tip60 was detected using western blotting (anti-HA antibody). Original immunoblot images for Fig. 3 are shown in Supplementary Fig. S10 . ( b ) Schematic representation of the five high confidence (filled circles) and one lower confidence (open circle) ubiquitination sites in Tip60 identified using MS/MS. ( c ) HEK293T cells were transfected with wild-type HA-tagged Tip60 expression construct or the 41 KR mutant together with histidine-tagged ubiquitin (His-ubi) and treated with MG132 (3 μM). Ubiquitinated Tip60 was detected as described under b . ( d ) HEK293T cells were transfected with HA-Tip60 expression vector with or without myc-USP7 expression vector and with or without his-tagged ubiquitin expression vector in the absence or presence of MG132, as indicated. Cells were lysed, ubiquitinated proteins were isolated by Ni-NTA purification and immunoreactive proteins were detected on western blots by anti-HA, anti-Tip60 and anti-myc antibodies. ( e ) Ubiquitinated HA-Tip60 and HA-PPARγ were produced as described in a , eluted from the Ni-NTA beads with imidazole and incubated with recombinant USP7 enzyme. Tip60 and PPARγ were detected using western blot analysis (anti-HA antibody). ( f ) HA-Tip60 expression vector was cotransfected with empty vector or USP7 expression vector in 911 cells. Cells were treated with cycloheximide (30 ng ml −1 ), collected at different time points and subjected to western blot analysis. ( g ) Mature 3T3-L1 adipocytes were subjected to RNAi-mediated knockdown with control or USP7-specific oligonucleotides. Cell lysates were subjected to western blot analysis using antibodies against USP7, Tip60 and tubulin. Full size image To investigate whether USP7 can deubiquitinate Tip60, we first performed ubiquitination experiments in the absence or presence of USP7 in living cells. As shown in Fig. 3d , inhibition of the proteasome by MG132 resulted in the accumulation of ubiquitinated forms of Tip60. Co-expression of USP7 clearly reduced the levels of ubiquitinated Tip60. To exclude the possibility that USP7 affected Tip60 protein stability indirectly, we performed in vitro deubiquitination assays. Recombinant USP7 clearly reduced the levels of Tip60 polyubiquitination ( Fig. 3e ). Importantly, recombinant USP7 displayed substrate specificity in vitro , as PPARγ, a well-established ubiquitinated protein [26] , was not affected by USP7 activity ( Fig. 3e ). Next, we examined the effect of USP7 on Tip60 protein levels. For this, Tip60 was expressed alone or together with USP7, and cells were treated for different periods of time with the protein translation inhibitor cycloheximide. In the absence of USP7, the amount of the Tip60 protein gradually decreased in time ( Fig. 3f ). Co-expression of USP7 significantly increased the steady-state level of Tip60, and higher Tip60 protein expression levels were observed at all time points ( Fig. 3f ). Finally, to examine the role of USP7 in regulating endogenous Tip60 protein levels, USP7 was knocked down in mature 3T3-L1 adipocytes, using the most effective siRNA oligonucleotide against USP7 (no. 12; Fig. 1e ). USP7 knockdown resulted in a marked reduction in the Tip60 protein ( Fig. 3g ) but not in mRNA expression ( Supplementary Fig. S4 ). Taken together, these data show that USP7-mediated deubiquitination regulates Tip60 protein levels. Tip60 and USP7 regulate common target genes Having established that USP7 interacts with and deubiquitinates Tip60 ( Figs 2 and 3 ), it was investigated whether Tip60 and USP7 are functionally linked to adipocyte differentiation. As knockdown of USP7 may indirectly reduce Tip60 levels by inhibiting adipogenesis ( Fig. 1d,e ) [17] , analysis of the transcriptome under these conditions is likely to reflect the differentiation status rather than gene regulation through Tip60 and/or USP7. We therefore performed knockdown experiments in differentiated 3T3-L1 adipocytes. On the basis of previous experiments, the most effective siRNA oligonucleotides against Tip60 (no. 2; (ref. 17 )) and USP7 (no. 12; Figs 1e and 3g ) were used. Treatment of mature 3T3-L1 adipocytes with these oligonucleotides resulted in ~80% reduced expression of Tip60 and USP7 ( Supplementary Fig. S4 ). Microarray analysis revealed that the expression of 1646 and 171 genes were altered after the knockdown of Tip60 or USP7, respectively ( Fig. 4a ). A highly significant overlap ( P -value 4.46 × 10 −40 ) was found between the data sets, consisting of 78 genes that are altered upon Tip60 and USP7 knockdown and these genes were either upregulated (20 genes) or downregulated (58 genes). Microarray results were validated using quantitative RT–PCR ( Supplementary Fig. S5 ). As USP7 regulates Tip60 protein levels ( Fig. 3 ), knockdown of USP7 would be predicted to have the same effect as the knockdown of Tip60. Indeed, knockdown of Tip60 or USP7 altered the expression of 76 of the 78 commonly affected genes in the same direction ( Fig. 4b ). As >45% of the USP7-regulated genes are also regulated by Tip60 (78 out of the 171), our findings suggest that Tip60 is an important mediator of gene regulation by USP7. USP7 seems to have a less dominant role in Tip60-mediated gene regulation, as the proportion of Tip60 target genes that is also regulated by USP7 is much smaller (78 out of 1,646). To identify the function(s) of the Tip60–USP7 target genes, we preformed Ingenuity Pathway Analysis with both complete transcriptome data sets. The pathway most clearly affected is the cell cycle, with the majority of genes being downregulated upon the knockdown of Tip60 or USP7 ( Fig. 4c and Supplementary Figs S6 and S7 ). Interestingly, a significant proportion of the commonly regulated genes (underlined genes in Fig. 4b ), including the genes encoding cell division cycle 20 (Cdc20) and Aurora kinase A (Aurka), display cycling expression patterns during adipogenesis with high expression in preconfluent cells (day −2), a drop in expression upon reaching confluency (day 0), followed by a rise in expression around days 1–2, after which expression drops again ( Fig. 4d ) [27] . Knockdown of USP7 or Tip60 blunted the cycling expression pattern of Cdc20 and Aurka, confirming that the expression of these genes is regulated by Tip60 and USP7 ( Fig. 4d ). Chromatin immunoprecipitation analysis revealed that Tip60 is recruited to the Cdc20 and Aurka genes upon differentiation. Tip60 could not be detected on an arbitrary intergenic region, which served as a negative control ( Fig. 4e ). 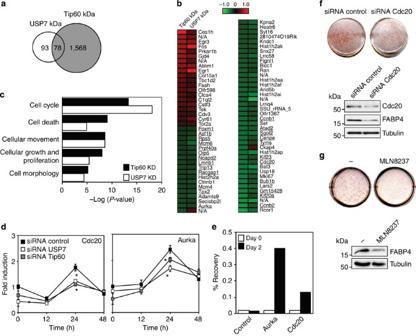Figure 4: A Tip60–USP7 gene regulation pathway in 3T3-L1 adipogenesis. (a) Mature 3T3-L1 adipocytes were subjected to RNAi-mediated knockdown with control, USP7- or Tip60-specific oligonucleotides. mRNA expression was assessed with microarray analysis. Shown are the number of genes with aP<0.05 after FDR correction and 5,000 permutations, which were >1.14-fold changed after the knockdown of Tip60 or USP7 compared with control cells. Data were obtained from experiments performed in quadruplicate. (b) Heat map showing log 2 fold change in gene expression after the knockdown of TIP60 or USP7 in differentiated 3T3-L1 cells. Red indicates increased gene expression compared with the control siRNA treatment, whereas green indicates decreased expression. (c) Biological functions were identified with the functional analysis of the Ingenuity Pathway Analysis. Only the top six significantly regulated molecular and cellular functions are shown. The –log (P-value) shown on thexaxis was calculated by Fisher’s exact test. Functions are included when Fisher’s exactP-value <0.05. (d) 3T3-L1 cells, transfected with control, Tip60 or USP7 siRNA oligonucleotides, were subjected to differentiation conditions. At different time points, mRNA expression levels of Cdc20 and Aurka were analysed using quantitative RT–PCR. Data are presented as mean (n=4) after correction forTFIIBexpression. Error bars represent the s.d., asterisks (*) indicate statistically significant differences (Student’st-test;P<0.05). (e) ChIP-PCR for Tip60 was performed in 3T3-L1 cells (days 0 and 2 of differentiation) with primers located near the TSS of theCdc20andAurkagenes. As a negative control, an intergenic region on chromosome 15 was used. Results are indicated as % of immunoprecipitated chromatin compared with the input. (f) 3T3-L1 cells, transfected with either control or Cdc20 siRNA oligonucleotides, were subjected to differentiation conditions. On the day 6 of differentiation, cells were fixed and stained for triglycerides using Oil-red-O. Pictures are representative for three independent experiments. Cell lysates were subjected to western blot analysis using antibodies against Cdc20, FABP4 and tubulin. Original immunoblot images forFig. 4are shown inSupplementary Fig. S11. (g) 3T3-L1 cells were treated with vehicle or the Aurka-specific chemical inhibitor MLN8237 (2 μM) from day 0 of differentiation onwards. Differentiation was analysed as described underf. Figure 4: A Tip60–USP7 gene regulation pathway in 3T3-L1 adipogenesis. ( a ) Mature 3T3-L1 adipocytes were subjected to RNAi-mediated knockdown with control, USP7- or Tip60-specific oligonucleotides. mRNA expression was assessed with microarray analysis. Shown are the number of genes with a P <0.05 after FDR correction and 5,000 permutations, which were >1.14-fold changed after the knockdown of Tip60 or USP7 compared with control cells. Data were obtained from experiments performed in quadruplicate. ( b ) Heat map showing log 2 fold change in gene expression after the knockdown of TIP60 or USP7 in differentiated 3T3-L1 cells. Red indicates increased gene expression compared with the control siRNA treatment, whereas green indicates decreased expression. ( c ) Biological functions were identified with the functional analysis of the Ingenuity Pathway Analysis. Only the top six significantly regulated molecular and cellular functions are shown. The –log ( P -value) shown on the x axis was calculated by Fisher’s exact test. Functions are included when Fisher’s exact P -value <0.05. ( d ) 3T3-L1 cells, transfected with control, Tip60 or USP7 siRNA oligonucleotides, were subjected to differentiation conditions. At different time points, mRNA expression levels of Cdc20 and Aurka were analysed using quantitative RT–PCR. Data are presented as mean ( n =4) after correction for TFIIB expression. Error bars represent the s.d., asterisks (*) indicate statistically significant differences (Student’s t -test; P <0.05). ( e ) ChIP-PCR for Tip60 was performed in 3T3-L1 cells (days 0 and 2 of differentiation) with primers located near the TSS of the Cdc20 and Aurka genes. As a negative control, an intergenic region on chromosome 15 was used. Results are indicated as % of immunoprecipitated chromatin compared with the input. ( f ) 3T3-L1 cells, transfected with either control or Cdc20 siRNA oligonucleotides, were subjected to differentiation conditions. On the day 6 of differentiation, cells were fixed and stained for triglycerides using Oil-red-O. Pictures are representative for three independent experiments. Cell lysates were subjected to western blot analysis using antibodies against Cdc20, FABP4 and tubulin. Original immunoblot images for Fig. 4 are shown in Supplementary Fig. S11 . ( g ) 3T3-L1 cells were treated with vehicle or the Aurka-specific chemical inhibitor MLN8237 (2 μM) from day 0 of differentiation onwards. Differentiation was analysed as described under f . Full size image To address the importance of commonly regulated genes such as Cdc20 and Aurka in adipogenesis, their expression and activity were inhibited, respectively. Knockdown of Cdc20 resulted in reduced differentiation as assessed by Oil-Red-O staining and FABP4 expression ( Fig. 4f ), whereas treatment with the Aurka-specific chemical inhibitor MLN8237 also reduced adipogenesis ( Fig. 4g ). Taken together, these data indicate that Tip60–USP7 target genes have an important role in adipogenesis. Tip60 and USP7 regulate early adipogenesis As 3T3-L1 cells undergo two sequential rounds of mitosis between day 0 and day 2 of differentiation, a process called MCE, and as the common Tip60–USP7 target gene set was enriched for cell cycle genes ( Fig. 4c ), we examined whether Tip60 and USP7 regulate the early steps in adipogenesis. First, an inhibitor that is active against a broad range of DUBs was added at different time points during 3T3-L1 differentiation ( Fig. 5a,b (ref. 28 )). The DUB inhibitor most clearly reduced adipogenesis when added at early time points (day 0–1), whereas the effects were less pronounced at later stages ( Fig. 5c,d ). These findings suggest that USP7 (and the low molecular weight DUB; Fig. 1b ) predominantly affects early adipogenesis. 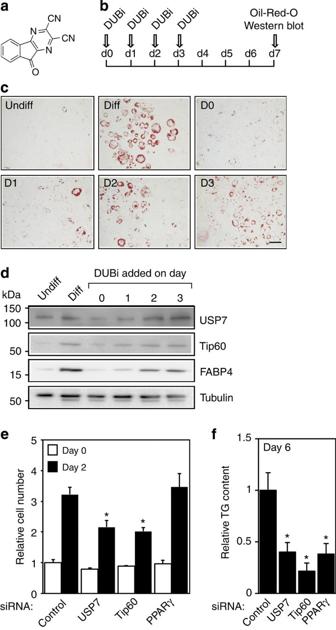Figure 5: Tip60–USP7 regulates early adipogenesis. (a) Structure of the DUB inhibitor. (b) Schematic presentation of the DUB inhibitor (DUBi) treatment during 3T3-L1 differentiation. (c) 3T3-L1 cells were treated with the DUB inhibitor (2 μM) or vehicle during differentiation, as presented inb. Differentiation was assessed with Oil-red-O staining. Scale bar, 50 μm. (d) 3T3-L1 cells were treated with the DUB inhibitor (2 μM) or vehicle during differentiation, as presented in (b). Cell lysates were subjected to western blot analysis using antibodies against USP7, Tip60, FABP4 and tubulin. Original immunoblot images forFig. 5are shown inSupplementary Fig. S12. (e) 3T3-L1 cells were subjected RNAi-mediated knockdown of genes indicated and induced to differentiate into adipocytes. Cell numbers were determined on days 0 and 2, and the relative cell number was plotted. Data are presented as mean (n=4). Error bars represent the s.d., asterisks (*) indicate statistically significant differences (Student’st-test;P<0.05). (f) 3T3-L1 cells were subjected to RNAi-mediated knockdown of genes as described ine, and triglyceride content was determined on the day 6 of differentiation. Data are presented as mean (n=3). Figure 5: Tip60–USP7 regulates early adipogenesis. ( a ) Structure of the DUB inhibitor. ( b ) Schematic presentation of the DUB inhibitor (DUBi) treatment during 3T3-L1 differentiation. ( c ) 3T3-L1 cells were treated with the DUB inhibitor (2 μM) or vehicle during differentiation, as presented in b . Differentiation was assessed with Oil-red-O staining. Scale bar, 50 μm. ( d ) 3T3-L1 cells were treated with the DUB inhibitor (2 μM) or vehicle during differentiation, as presented in ( b ). Cell lysates were subjected to western blot analysis using antibodies against USP7, Tip60, FABP4 and tubulin. Original immunoblot images for Fig. 5 are shown in Supplementary Fig. S12 . ( e ) 3T3-L1 cells were subjected RNAi-mediated knockdown of genes indicated and induced to differentiate into adipocytes. Cell numbers were determined on days 0 and 2, and the relative cell number was plotted. Data are presented as mean ( n =4). Error bars represent the s.d., asterisks (*) indicate statistically significant differences (Student’s t -test; P <0.05). ( f ) 3T3-L1 cells were subjected to RNAi-mediated knockdown of genes as described in e , and triglyceride content was determined on the day 6 of differentiation. Data are presented as mean ( n =3). Full size image Next, the role of Tip60 and USP7 on MCE was addressed more directly using RNAi-mediated knockdown experiments. In agreement with a previous report [2] , 3T3-L1 cells underwent two rounds of mitosis, resulting in an almost fourfold increase in cell number at 48 h ( Fig. 5e ). Both TIP60 and USP7 knockdown impaired MCE, as the number of cells on day 2 was significantly lower than control cells in both cases ( Fig. 5e ). Terminal differentiation, as assessed by quantification of triglyceride storage on day 6, was also impaired by the knockdown of Tip60 or USP7 ( Fig. 5f ), underscoring the importance of MCE for efficient 3T3-L1 adipogenesis. As a control, knockdown of PPARγ was performed, which did not affect MCE ( Fig. 5e ) but still inhibited terminal differentiation ( Fig. 5f ). Taken together, our findings have revealed deubiquitination of a transcriptional coregulator as a key mechanism in the regulation of early adipogenesis. Accumulating evidence indicates that the PTM of transcriptional coregulators presents an important mechanism to regulate fundamental cellular processes. Most studies have focused on modifying enzymes; however, demodification may have an equally important role in balancing the transcriptional output. Here we show a direct connection between the transcriptional coregulator Tip60, a histone acetyltransferase and the deubiquitinase USP7. These two proteins are broadly expressed, fulfil multiple roles in fundamental cellular processes and are both essential for embryonic development in mice [11] , [12] , [29] . Our data show that USP7 is an essential DUB in adipogenesis and reveal the underlying mechanisms to be deubiquitination and stabilization of Tip60. Our data indicate that enzymatic activity, rather than expression of the USP7 protein, is regulated during adipogenesis. Two molecular mechanisms, which are not mutually exclusive, have been described that can regulate USP7 activity: interaction with specific proteins and PTM. Studies in D. melanogaster and human cells found the metabolic enzyme GMP synthase to stimulate the ability of USP7 to deubiquitinate histone H2B [30] , [31] , [32] , whereas the TSPYL5 protein can inhibit the activity of USP7 towards p53 in mammalian cells [33] . Besides these two proteins, Sowa et al . [34] identified >30 additional USP7-interacting proteins using a global proteomic analysis. In addition, USP7 is subjected to ubiquitination [35] , [36] neddylation [35] and phosphorylation [36] , [37] —PTMs that could all potentially regulate the activity of USP7. Future studies are required to establish whether USP7 activity is regulated through protein–protein interactions, PTM or both mechanisms in adipogenesis. Several lines of evidence suggest that a dominant role of the Tip60–USP7 gene regulation pathway lies in the early stages of adipogenesis. First, the major changes in Tip60 protein expression occur during the first days of differentiation ((ref. 17 ), present study). Second, a significant proportion of the genes downregulated after the knockdown of either Tip60 or USP7 are mainly involved in mitotic cell cycling, and Tip60 has been shown to interact with mitotic regulators such as Plk1 and cyclin B1 (ref. 38 ). Third, knockdown of Tip60 or USP7 inhibited the two rounds of mitosis observed during MCE, an essential early step in 3T3-L1 adipogenesis. Finally, our transcriptome analysis revealed very few ‘late’ adipocyte genes to be critically regulated by Tip60 and/or USP7 ( Fig. 4b ), despite the fact that Tip60 is recruited to the Fabp4 , Plin1 (Perilipin) and Pparg promoters in mature 3T3-L1 adipocytes [17] , [18] . Taken together, these findings suggest that the critical role of Tip60–USP7 adipogenesis may be the regulation of MCE (days 0–2), whereas these proteins may be redundant for the maintenance of the adipogenic phenotype. It is tempting to speculate that Tip60 is recruited to its target genes by one of the transcription factors that is critical for the early steps in adipogenesis, such as CCAAT enhancer-binding protein β (ref. 3 ). However, our microarray analysis data did not clearly indicate that the Tip60-regulated genes were controlled by a common transcription factor. It should be noted that the NuA4/Tip60 complex may also be recruited to target genes through alternative mechanisms, such as H3 lysine 4 trimethylation [39] , histone acetylation [40] and RNA polymerase II phosphorylation [41] . Both Tip60 and USP7 have been identified as critical regulators of fundamental cellular processes, such as proliferation, apoptosis and differentiation. For example, Tip60 acetylates p53 at lysine 120, a modification that modulates the decision between cell cycle arrest and apoptosis [42] , [43] , whereas USP7 is involved in the same processes, as it functions as a deubiquitinase of p53 itself, its E3 ligase mdm2 (ref. 22 ) and Tip60. USP7 and Tip60 share another common target, DNMT1, which maintains DNA methylation patterns after cellular replication. Whereas USP7 stabilizes DNMT1 and facilitates cell cycle progression, Tip60 acetylates DNMT1 and promotes the degradation of DNMT1 by its E3 ligase UHRF1 (ref. 44 ). Besides having critical roles in proliferation and apoptosis, both Tip60 and USP7 have recently been implicated in cellular differentiation. Tip60 depletion in Caenorhabditis elegans results in premature cell cycle exit and differentiation of one particular cell type, the vulval cells [45] . Second, Tip60 was shown to be essential for the maintenance of embryonic stem cell identity, probably through regulation of the cell cycle and proliferation and by repressing the expression of multiple differentiation genes [39] . Interestingly, Tip60 knockdown had only very modest effects on MEF cell cycle distribution and proliferation. USP7 has also been implicated in the regulation of cell differentiation. By deubiquitinating the transcription factor REST, USP7 plays a critical role in the maintenance of neural progenitor cells [46] . Whereas these studies indicate that Tip60 and/or USP7 are important to maintain cells in an undifferentiated state, the differentiation of 3T3-L1 adipocytes and human primary adipocytes critically depends on Tip60 (refs 17 , 47 ), on the Brd8 and p400 proteins, which are also part of the NuA4/Tip60 complex [18] , and on USP7 (current study). Taken together, current evidence therefore suggests that Tip60 and USP7can both inhibit and stimulate proliferation, apoptosis and differentiation, depending on the cellular context. Unravelling the function of Tip60 and USP7 by identifying their upstream regulators and downstream effectors will therefore not only contribute to our understanding of adipogenesis but may also help to unravel the fundamental link(s) between cell cycle control and differentiation. While this manuscript was under review, Dar et al . [48] reported that USP7 can interact with and deubiquitinate Tip60, and they show the stabilization of Tip60 to be required for an effective p53-dependent apoptotic pathway. Together with our current findings in adipogenesis, these studies underscore the relevance of USP7-mediated Tip60 stabilization in multiple independent biological pathways. Antibodies and reagents The following antibodies were used, with the dilutions used for WB: anti-Tip60 (sc-5725 and sc-5727; WB 1:400), anti-USP7 (sc-22848; WB 1:1,000), anti-FABP4 (sc-18661; WB 1:1,000), anti-Cdc20 (sc-8358; WB 1:400) and anti-myc (sc-40; WB 1:1,000), from Santa Cruz Biotechnology (Santa Cruz, CA, USA), anti-Tip60 (07-038) from Millipore (Billerica, MA, USA), anti-Tip60 (DR1041; WB 1:1,000) from EMD4 biosciences (Gibbstown, NJ, USA), anti-USP7 (A300-033A; WB 1:1,000) from Bethyl Laboratories (Montgomery, TX, USA), anti-mouse-HRP (1858413; 1:10,000) from Pierce Biotechnologies (Rockford, IL, USA), anti-HA (H9658; WB 1:1,000), anti-actin (A5060; WB 1:1,000), anti-tubulin (T9026; WB 1:1,000) and anti-goat-HRP (A9552; WB 1:10,000) from Sigma-Aldrich (St Louis, MO, USA). Anti-HA (A2095) or anti-Myc-conjugated agarose beads (A7470) were from Sigma-Aldrich. True blot Rabbit IgG beads (00-8800) were from Bioscience (San Diego, CA, USA) and True blot secondary anti-rabbit antibody (18-8816-31;WB 1:10,000) was from Pierce Biotechnologies. Antibody dilutions for applications other than WB are given in the respective sections. The vinyl methyl ester HA-DUB probe (HAUbVME) was generated by chemical ligation of HAUb75-MESNa and glycine vinyl methylester (VME) and was purified using cation-exchange chromatography [20] , and the DUB inhibitor (DUBi) was prepared by reaction between ninhydrin and diaminomaleonitrile [28] . The Aurka-specific chemical inhibitor MLN8237 was from Selleck Chemicals (Houston, TX, USA). Plasmids and siRNAs pCDNA-HA-Tip60 (ref. 16 ) and pCL-Myc-USP7 (ref. 49 ) were kind gifts of D. Trouche and M. Maurice, respectively. pGEX2T-USP7 was a kind gift of J. Bartek and J. Lukas [50] . Tip60 deletion constructs were generated by standard cloning procedures [51] . Control siRNA oligonucleotides (D-001810-10), pooled siRNA duplexes against mAurka (L-065109-00) and Cdc20 (L-048688-00) and individual siRNA duplexes against mUSP7 (LQ-052244-01) and mTIP60 (LQ-057795-01) were from Dharmacon (Lafayette, CO, USA). MG132 (474790) was from EMD4 Biosciences. Cell culture and differentiation assays Human embryonic kidney 293T cell line (HEK293T) and human embryonic retina 911 cell line were maintained in DMEM Glutamax (Invitrogen, Carlsbad, CA, USA) containing 10% fetal calf serum (Invitrogen), penicillin and streptomycin (Invitrogen) and transfected using the CaPO4 method [17] , [52] . The 3T3-L1 cell line was cultured in the same media with 10% bovine serum (Invitrogen). Differentiation was induced by growing cells to confluency, and after 2 days the cells were incubated with culture medium containing dexamethasone (250 nM), IBMX (500 μM), insulin (170 nM) and rosiglitazone (2.5 nM) for 2 days. On day 3, medium was changed for culture medium supplemented with insulin (170 nM) and rosiglitazone (2.5 nM) and left for 2–7 days [17] , [52] . Differentiation was analysed with Oil-red-O staining and WB [17] , [52] , using anti-Tip60 (sc-5725 and DR1041) and anti-USP7 (A300-033A) antibodies. Undifferentiated cells were transfected with siRNA oligonucleotides using RNAiMAX transfection (Invitrogen) [17] . siRNA oligonucleotides were introduced into differentiated 3T3-L1 cells with Amaxa technology using buffer L [53] . Triglycerides were determined using the Infinity Triglycerides kit (TR 2291-030; Thermo Electron, Louisville, CO, USA) according to the manufacturer’s instructions. Results are expressed as TG content relative to control samples and as means ±s.d. Differences between the means were statistically assessed by a Student’s t -test in which the limit of significance was set as P <0.05. DUB activity assays and deubiquitination assays To analyse DUB activity in 3T3-L1 cells, lysates were made in RIPA buffer and cleared using centrifugation. For DUB activity in mouse tissues, epidydimal WAT and interscapular BAT were isolated from wild-type male C57 Bl/6 mice, and lysates were made with M-PER Mammalian Protein Extraction Reagent (Thermo Fisher Scientific, Etten-Leur, The Netherlands) according to the manufacturer’s instructions. Lysates were incubated with DUB probe (0.1 μg probe per 20 μg cell lysate) for 1 h at 37 °C (ref. 20 ). Samples were directly subjected to western blot analysis, or DUB activity was first immunoprecipitated using a monoclonal HA-conjugated-agarose antibody. For in vivo (de)ubiquitination assays, cells were transfected with HA-Tip60 and/or myc-USP7 and His-ubi expression plasmids. Twenty-four hours after transfection, cells were incubated o/n with MG132 (3 μM) and lysed, and his-tagged proteins were isolated by purification on Ni-NTA agarose beads [49] , [54] . Precipitates were subjected to WB. For in vitro deubiquitination assays, his-tagged polyubiquitinated HA-Tip60 was isolated as described above. Recombinant human His6-USP7 (E-519; Boston Biochem, Boston, MA, USA) was added to the substrates for 1 h at 37 °C in deubiquitination buffer (50 mM Tris PH 7.4, 150 mM NaCl, 10 mM DTT, 5 mM MgCl 2 ). Reactions were stopped by adding 2 × SDS sample buffer and analysed using WB. Mass spectrometry analysis Proteins were separated using SDS–PAGE on 4–12% NuPAGE gels (Invitrogen) and stained with Simply Blue Safestain (Invitrogen). Bands were excised from gel, reduced with dithiothreitol, alkylated with iodoacetamide and digested with trypsin (Roche Applied Science, Almere, The Netherlands) [55] . Samples were subjected to nanoflow LC (Eksigent, Dublin, Ireland) using C 18 reverse phase trap columns (Phenomenex, Utrecht, The Netherlands; column dimensions 2 cm × 100 μm, packed in-house) and subsequently separated on C 18 analytical columns (Reprosil; column dimensions, 20 cm × 50 μm; packed in-house) using a linear gradient from 0 to 40% B (A=0.1 M acetic acid; B=95% (v/v) acetonitrile, 0.1 M acetic acid) in 60 min and at a constant flow rate of 150 nl min −1 . Column eluate was directly coupled to a LTQ-Orbitrap-XL mass spectrometer (Thermo Fisher Scientific, Breda, The Netherlands) operating in positive mode, using Lock spray internal calibration. Data were processed and subjected to database searches using MASCOT software (Matrix Science, Boston, MA, USA) against Swiss Prot and non-redundant NCBI database, with a 10 p.p.m. mass tolerance of precursor and 0.8 Da for the fragment ion. Immunoprecipitation assays Immunoprecipitation experiments were performed using anti-HA- or anti-Myc-conjugated agarose (30 μl slurry/sample [17] ). Precipitates were subjected to WB using antibodies against myc and HA tags, respectively. Endogenous co-immunoprecipitation experiments on differentiated 3T3-L1 cells were performed similarly, using anti-Tip60 (DR1041) antibody (5 μg per sample), True blot Rabbit IgG beads and True blot secondary anti-rabbit antibody (Pierce Biotechnologies). Immunofluorescence microscopy and PLA For immunofluorescence staining, 3T3-L1 cells were plated on glass coverslips and differentiated for 5 days. Subsequently, cells were fixed with 4% paraformaldehyde (20′, RT) and permeabilized in phosphate-buffered saline (PBS) supplemented with 0.5% Triton (10′). After 30′ incubation in blocking buffer, cells were stained with primary antibodies (anti-Tip60 (DR1041) and anti-USP7 (sc-22848); both 1:200 dilution) for 2 h at room temperature, and then incubated with secondary fluorochrome-conjugated antibodies (1:300 dilutions). After several washes, coverslips were incubated with Nile Red and Hoechst, washed with PBS, mounted in Mowiol and analysed with an LSM710 Met confocal microscope (Carl Zeiss, Jena, Germany). PLA detection was performed using the Duolink II kit (Olink bioscience, Uppsala, Sweden). In short, differentiated 3T3-L1 cells were enabled to adhere to coverslips and subsequently washed with PBS and fixed with 4% formaldehyde for 20 min. Afterwards, the samples were permeabilized with 0.2% triton X-100 for 5 min and then incubated for 30 min with blocking buffer (10% normal human serum in PBS). After blocking, cells were incubated O/N at 4 °C with anti-Tip60 antibody (07-038) and anti-USP7 antibody (sc-22848) in blocking buffer containing 10% normal human serum. Cells were washed three times with PBS, followed by PLA according to the manufacturer’s protocol. Coverslips were mounted and analysed as described above. GST-pull-down assays Recombinant Tip60 construct in the pCDNA3 expression vector was transcribed and translated in vitro in reticulolysate in the presence of [ 35 S]-methionine according to the manufacturer’s protocol (TNT T7 Quick Coupled Transcription/Translation Kit; Promega, Leiden, The Netherlands). Rosetta pLysS competent bacteria (EMD4 Biosciences) were transformed with GST-USP7 expression plasmid [50] . GST fusion proteins were purified on glutathione- S -sepharose beads [52] and incubated with [ 35 S]-labelled protein in NETN buffer (20 mM Tris pH 8.0, 400 mM NaCl, 1 mM EDTA, 0.5% NP40) containing protease inhibitors (Complete; Roche Applied Science). Samples were subsequently washed and subjected to SDS–PAGE. Gels were enhanced with Amplify (Amersham), dried and visualized using fluorography. Chromatin immunoprecipitation PCR analysis For chromatin preparation, 10 8 3T3-L1 (2 days of differentiation) were crosslinked with 2 mM disuccinimidyl glutarate (Thermo Fisher Scientific) and 1% formaldehyde as previously described [56] ; nuclei were isolated in lysis buffer (10 mM Tris-Cl pH 7.5, 10 mM NaCl, 3 mM MgCl 2 , 0.5% Igepal) and lysed in pre-immunoprecipitation buffer (10 mM Tris, 10 mM NaCl, 3 mM MgCl 2 and 1 mM CaCl 2 ). Chromatin was sheared using a Bioruptor (Diagenode, Denville, USA), and chromatin was precipitated with 5 μg anti-Tip60 antibody (sc-5727; 3 μg per sample) and protG-sepharose beads (Sigma-Aldrich). De-crosslinked and precipitated chromatin was dissolved in 100 μl water, and 5 μl of DNA solution was used for qPCR analysis. The primers used for qPCR were Cdc20 forward primer 5′-GGGATTTCCTTCCAAATGCT-3′ and reverse primer 5′-TCATTGGCTCCTTCAAAACC-3′; Aurka forward primer 5′-AAACGGATAGGGAAGGCTGT-3′ and reverse primer 5′-CCCATTCCCACAAGAACCTA-3′; intergenic region on mouse chromosome 15 forward primer 5′-TGGTAGCCTCAGGAGCTTGC-3′ and reverse primer 5′-ATCCAAGATGGGACCAAGCTG-3′. RNA isolation followed by microarray analysis and qRT–PCR Differentiated 3T3-L1 cells were transfected with the Amaxa technology as described above. Two days after transfection, cells were washed twice with PBS and lysed in 0.5 ml Trizol (Invitrogen). Samples were incubated at room temperature for 5′; 0.1 ml chloroform was added, vortexed and centrifuged for 10 min at 8,000 r.p.m. at 4 °C. The pellet was washed with 70% ethanol and dissolved in water. DNAse treatment and purification were performed with RNeasy kit (Qiagen, Venlo, The Netherlands). Microarrays used were Mouse Whole Genome Gene Expression Microarrays V1 (Agilent Technologies, Belgium) representing 41174 Mus musculus 60-mer probes in a 4 × 44 K layout. RNA amplifications and labelling were performed [57] on an automated system (Caliper Life Sciences NV/SA, Belgium) with 3 μg total RNA from each sample. Hybridizations were carried out on an automated hybridization station (HS4800PRO system with QuadChambers; Tecan Benelux B.V.B.A.) using 1,000 ng labelled cRNA per channel according to van de Peppel et al . [58] Hybridized slides were scanned on an Agilent scanner (G2565BA) at 100% laser power and 30% PMT. After automated data extraction using Imagene 8.0 (BioDiscovery), printtip Loess normalization was performed [59] on mean spot intensities. Data were analysed using MAANOVA [60] . In a fixed effect analysis, sample, array and dye effects were modelled. P -values were determined using a permutation F2-test, in which residuals were shuffled 5,000 times globally. Genes (based on unique ENSMUSG gene IDs) with P <0.05 after the determination of false discovery rate (FDR) were considered significantly changed. A cutoff fold change greater than ±1.14 was used. Hypergeometric testing was performed to identify significance of overlap. Microarray data were analysed with Ingenuity Pathway Analysis (Ingenuity Systems, www.ingenutiy.com ). Functional analysis identified biological functions that were differentially expressed between knockout and wild-type cells. Genes with P <0.05 after FDR that met the cutoff fold change of more than ±1.14 and that were associated with a biological function in the Ingenuity Pathway Knowledge Base were included for the analysis. Fisher’s exact test was used to calculate a P -value for each biological function, and functions were considered to be differentially expressed between genotypes when the Fisher’s exact P -value <0.05. In addition, biological interaction networks for Tip60- and USP7-regulated genes were identified. A statistical likelihood approach was used to identify the significance of the generated networks. Microarray data have been submitted to ArrayExpress (E-TABM-1145) and GEO (GSE28587). For qRT–PCR analysis, three independent samples of total RNA were reverse-transcribed with SuperScript III reverse transcriptase (Invitrogen). Gene expression levels were determined using quantitative real-time PCR with the MyIq cycler (Bio-Rad) using SYBR-green (Bio-Rad) and normalized to TFIIb expression. The primers used were TFIIb forward primer 5′-TCCTCCTCAGACCGCTTTT-3′ and reverse primer 5′-CCTGGTTCATCATCGCTAATC-3′; Cdc20 forward primer 5′-GCTCAAAGGACACACAGCAC-3′ and reverse primer 5′-GCCACAACCGTAGAGTCTCA-3′; Asf1b forward primer 5′-CTGACGACCTGGAGTGGAAG-3′ and reverse primer 5′-AGGTGCAGGTGATGAGAACC-3′; Mcm4 forward primer 5′-GTCACACTGGGAGGGGTAAA-3′ and reverse primer 5′-CACTGGAGCCTTTTCCAGAC-3′; Egr1 forward primer 5′-CTGACCACAGAGTCCTTTTCTG-3′ and reverse primer 5′-GTTCAGGCCACAAAGTGTTG-3′; Fos forward primer 5′-CCAAGCGGAGACAGATCAACT-3′ and reverse primer 5′-TGGGCTGCCAAAATAAACTC-3′; Aurka forward primer 5′-CATGCTCCATCTTCCAGGAG-3′ and reverse primer 5′-AGGCATCCCCACTAGGAACT-3′. Results are expressed as mRNA expression relative to control samples and as means±s.d. Differences between the means were statistically assessed by a Student’s t -test in which the limit of significance was set as P <0.05. How to cite this article: Gao, Y. et al . Early adipogenesis is regulated through USP7-mediated deubiquitination of the histone acetyltransferase TIP60. Nat. Commun. 4:2656 doi: 10.1038/ncomms3656 (2013).